Metabolomic high-content nuclear magnetic resonance-based drug screening of a kinase inhibitor library Metabolism is altered in many highly prevalent diseases and is controlled by a complex network of intracellular regulators. Monitoring cell metabolism during treatment is extremely valuable to investigate cellular response and treatment efficacy. Here we describe a nuclear magnetic resonance-based method for screening of the metabolomic response of drug-treated mammalian cells in a 96-well format. We validate the method using drugs having well-characterized targets and report the results of a screen of a kinase inhibitor library. Four hits are validated from their action on an important clinical parameter, the lactate to pyruvate ratio. An eEF-2 kinase inhibitor and an NF-kB activation inhibitor increased lactate/pyruvate ratio, whereas an MK2 inhibitor and an inhibitor of PKA, PKC and PKG induced a decrease. The method is validated in cell lines and in primary cancer cells, and may have potential applications in both drug development and personalized therapy. Metabolism has a central role in many diseases and recent genome-wide reconstructions have defined the number of metabolic enzymes in the human genome and their relationships [1] . The large size and the connectivity of the metabolic network suggest that multiple controllers are needed for a robust control of its function and indeed metabolism is regulated within cells by large combinations of regulators, including transcription factors, microRNAs (miRs), allosteric effects of metabolites and signal transduction pathways. Therefore, there is a clear need for a well-characterized set of drugs and research tools that function on metabolism. To accelerate drug discovery, over the last decade, high-throughput screening (HTS) has gained widespread popularity in pharmaceutical companies and increasingly in academia to conduct a large number of biochemical, genetic or pharmacological tests [2] , [3] , [4] . Most screens monitor a single variable, often related to the action on a single target. Screening with a multivariate readout, also called high content screening (HCS), has recently become more popular, and might facilitate the identification of interventions for more complex phenotypes. Until now, HCS has been mainly associated with automated digital microscopy [3] , [4] , [5] . Using omic measurements for HCS would have the advantage of providing multivariate readouts more clearly linked to the drug targets and more easily amenable to network-based modelling and therefore to mechanistic insight. For example, a model could include the kinases targeted by kinase inhibitors (KIs), metabolic enzymes regulated by these kinases and the metabolites affected by these enzymes. We are not aware of any report of a drug library screen on mammalian cells that uses metabolomics. High-resolution NMR spectroscopy and mass spectrometry (MS) are the most common analytical platforms for the identification and quantification of intracellular and extracellular metabolites [6] , [7] , [8] , [9] , [10] , [11] . Regardless of sample volume and analytical techniques used, several crucial steps are required for separating the culture media from the cells, and extracting the intracellular metabolites using organic solvents [7] , [10] . Depending on the characteristics of the cells being extracted, the overall extraction process typically includes centrifugation steps, organic phase separation and lengthy drying procedures. The dried intracellular extract is then re-dissolved in solvents suitable for the analytical technique. A recent high-throughput metabolomic study has been applied to a 96-well plate to study the intracellular yeast metabolome [12] . To maximize the information contained in a multi-well plate, the authors have optimized cultivation, quenching and extraction of yeast pellets before chemical derivatization and subsequent gas chromatography/time of flight MS analysis. Although all the abovementioned approaches are extremely useful for obtaining clear and detailed information from both intra- and extra-cellular metabolism, they have not been optimized and used for the rapid preparation and metabolomic screening of hundreds of drug-treated mammalian cell samples. In this paper, we describe a high-resolution NMR-based method for screening the global metabolic changes induced by drug interventions in primary cells and cell lines performed in a 96-well plate format with a simple and rapid sample preparation. We first validated the screening method using both suspension and adherent carcinoma cell lines, and primary cells treated with a small number of drugs having well characterized targets. To validate this approach, we applied unsupervised multivariate statistical modelling and calculated the Z -factor value, a commonly used parameter for monitoring the quality of HTS assays [13] , [14] , [15] . Then, as a large screening application, we profiled the metabolomic response of cancer cells to a library of KIs. The development of a robust high-content metabolomic platform would be extremely valuable to accelerate the understanding of the in vitro and in vivo actions of drugs and aid their incorporation into therapeutic settings. Metabolomic NMR-based drug screening validation A crucial step in the development of a metabolomics screening method exploiting a NMR platform is to design a quick, simple, robust and reproducible sample preparation protocol. Here, we have developed a procedure for screening the response of a sub-selection of metabolites from cells seeded in a 96-well plate without a lengthy sample preparation. The cells of interest were seeded in a 96-well plate and treated with several drugs ( Fig. 1a ). 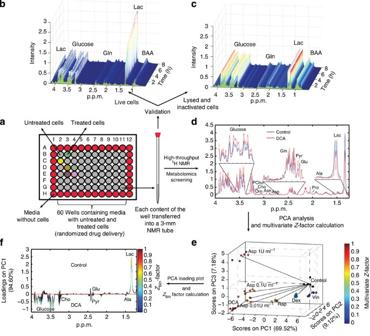Figure 1: Validation and workflow for NMR-based metabolomic drug screening. (a) The cells are seeded and treated in a 96-well plate. At the end of the 24 h treatment period, cells are lysed and their metabolism quenched by combined ultrasonication and by addition of SDS-d25. The content of the well is then transferred into a 3-mm NMR tube. To validate the quenching of any residual enzymatic activity, metabolic changes were monitored by NMR in live cells (b) and cells lysed and inactivated by addition of SDS-d25and ultrasonication (c). 1-D NMR spectra were acquired every 30 min for a total of 8 h. (d)1H-NMR spectra showing the metabolomic perturbations induced in CCRF-CEM cells after 24 h of drug treatment ((Dex, Rap, DCA, Vin) and three different doses of asparaginase (A1, 1 U ml−1; A01, 0.1 U ml−1; A001, 0.01 U ml−1)). Overlay of six replicate spectra (1.3–4 p.p.m. section) per treatment condition (with and without DCA treatment) highlights the degree of reproducibility. The metabolic changes detected determine a good separation between the different treatment groups, as shown in the 3-D scores plots (e), obtained from the PCA of the CPMG NMR spectra. Each treatment group is colour-coded according to the multivariateZ-factor value (colour bar) obtained by the pairwise PCA comparison of each drug treatment versus solvent control (Dex (Z=0.15), DCA (Z=0.91), Rap (Z=0.74), Vin (Z=−1.97), A1 (Z=0.91), A01 (Z=0.86), A001 (Z=0.84)). (f) PCA loadings plot and the superimposedZbin-values identify both the contribution and theZ-factor values of every bin of NMR spectra from the comparison of control and DCA intervention. (Lac, lactate; Ala, alanine; Pro, proline; Glu, glutamate; Pyr, pyruvate; Gln, glutamine; Asp, aspartate; Asn, asparagine; Orn, ornithine; Cho, choline; PCho, phosphocholine). To lyse the cells and immediately quench their metabolism we used the procedure detailed in the Methods section and in Figure 1 . Briefly, sodium dodecyl sulphate (SDS; final concentration 0.5% w/v) was added to each well of the 96-well plate and the cells (in medium and SDS) were immediately ultrasonicated by immersing the plate in an ice-cold sonicating water bath. The entire content of the well (endo- and exo-metabolome) was then transferred into a 3-mm NMR tube containing phosphate buffer and trimethylsilylpropionate-2,2,3,3-d4 (TMSP). This simple and rapid sample preparation was then followed by NMR spectra acquisition. The overall time for lysing the cells and quenching their enzymatic activity was approximately 5 min. Figure 1: Validation and workflow for NMR-based metabolomic drug screening. ( a ) The cells are seeded and treated in a 96-well plate. At the end of the 24 h treatment period, cells are lysed and their metabolism quenched by combined ultrasonication and by addition of SDS-d 25 . The content of the well is then transferred into a 3-mm NMR tube. To validate the quenching of any residual enzymatic activity, metabolic changes were monitored by NMR in live cells ( b ) and cells lysed and inactivated by addition of SDS-d 25 and ultrasonication ( c ). 1-D NMR spectra were acquired every 30 min for a total of 8 h. ( d ) 1 H-NMR spectra showing the metabolomic perturbations induced in CCRF-CEM cells after 24 h of drug treatment ((Dex, Rap, DCA, Vin) and three different doses of asparaginase (A1, 1 U ml −1 ; A01, 0.1 U ml −1 ; A001, 0.01 U ml −1 )). Overlay of six replicate spectra (1.3–4 p.p.m. section) per treatment condition (with and without DCA treatment) highlights the degree of reproducibility. The metabolic changes detected determine a good separation between the different treatment groups, as shown in the 3-D scores plots ( e ), obtained from the PCA of the CPMG NMR spectra. Each treatment group is colour-coded according to the multivariate Z -factor value (colour bar) obtained by the pairwise PCA comparison of each drug treatment versus solvent control (Dex ( Z =0.15), DCA (Z=0.91), Rap ( Z =0.74), Vin ( Z =−1.97), A1 ( Z =0.91), A01 ( Z =0.86), A001 ( Z =0.84)). ( f ) PCA loadings plot and the superimposed Z bin -values identify both the contribution and the Z -factor values of every bin of NMR spectra from the comparison of control and DCA intervention. (Lac, lactate; Ala, alanine; Pro, proline; Glu, glutamate; Pyr, pyruvate; Gln, glutamine; Asp, aspartate; Asn, asparagine; Orn, ornithine; Cho, choline; PCho, phosphocholine). Full size image To evaluate the robustness and reproducibility of this method in stopping the cellular enzymatic activity, we compared the effect of adding different concentrations of SDS (final concentration 0.01–2% w/v) on cell viability and ATP levels ( Supplementary Fig. S1 ). No enzymatic activity was detected upon addition of 0.1% SDS; however, we decided to exceed the critical micelle concentration of this detergent and use a final concentration 0.5% w/v to guarantee the complete quenching of cellular metabolism. To further validate these results, we monitored the metabolic variations in CCRF-CEM (non-adherent) samples by acquiring a series of NMR spectra every 30 min over a period of 8 h. We compared live cells ( Fig. 1b ), cells lysed using only ultrasonication ( Supplementary Fig. S2 ) and cells lysed and inactivated using combined 0.5% SDS-d 25 and ultrasonication ( Fig. 1c ). All the samples prepared using the combined SDS/ultrasonication method displayed no detectable metabolic alteration for the entire period of acquisition (8 h). On the contrary, metabolic changes (for example, glucose consumption and lactate production; Fig. 1a ; Supplementary Fig. S2 ) were observed for samples containing live or ultrasonicated cells (incomplete quenching process). Multivariate statistical modelling using principal component analysis (PCA) was also performed on the spectra acquired on live, lysed and on simultaneously lysed and inactivated cells ( Supplementary Fig. S3 ). The PCA plot shows important metabolic perturbation for live as well as lysed cells; the extremely tight grouping of the time-series NMR spectra acquired on samples of cells previously lysed and SDS-inactivated clearly demonstrates the absence of residual metabolic activity. Notably, the use of labelled SDS (98% SDS-d 25 ) minimizes the signal interference of the resonances arising from the detergent in the NMR analysis. The small signals deriving from residual unlabelled SDS were constant through all the samples, as the same amount of SDS was added to each well. Therefore, SDS does not interfere with NMR processing and multivariate analysis. A legitimate question might arise regarding the relative contribution of the intracellular metabolome to the NMR spectrum acquired on the well content, including both medium and the lysed cell metabolomes. To address this question we acquired NMR spectra on the entire content of the well (endo- and exo-metabolomes), the exometabolome, the endometabolome and medium ( Supplementary Fig. S4 ). The samples containing only the endometabolome were prepared by extracting PBS-washed cells from one well using the combined SDS/ultrasonication method. As expected, the major NMR signals arose from the extracellular metabolites; however, several signals arising from the intracellular metabolites were detected (for example, glutamate, choline, phosphocholine and so on). Similarly, in spectra acquired on samples containing both endo- and extracellular metabolomes, signals arising exclusively from the endometabolome and not overlapping with other extracellular resonances were clearly identified (for example, phosphocholine and glycerophosphocholine; Supplementary Fig. S4 ). To validate the robustness of the method across multiple 96-well plates, we applied PCA to 1 H-NMR spectra acquired on samples seeded with either solvent control or L -asparaginase in randomized positions within one plate as well as in different plates. No plate-to-plate variability was observed and further details are reported in Supplementary Fig. S5 . Metabolic changes induced by drug treatment in cell lines To evaluate the sensitivity of this method for monitoring metabolic perturbations induced by a 24-h drug treatment, we compared the metabolic changes of both suspension (human leukaemia cells, CCRF-CEM) and adherent mammalian carcinoma cell lines (human ovarian cancer cells, SKOV-3) in response to different drug treatments (dexamethasone (Dex), rapamycin (Rap), dichloroacetate (DCA), vincristine (Vin) and three different doses of L -asparaginase (A1, 1 U ml −1 ; A01, 0.1 U ml −1 ; A001, 0.01 U ml −1 )). For each cell line, we compared spectra acquired using three different 1 H NMR pulse sequences: One-dimensional (1-D) spectra ( Fig. 2a ), Carr-Purcell-Meiboom-Gill (CPMG) spin echo ( Fig. 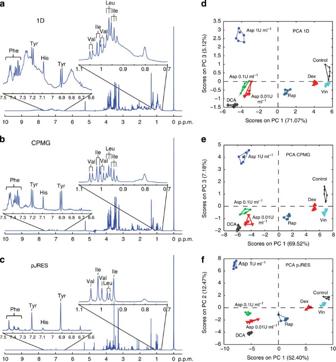Figure 2: Comparison of different NMR pulse sequences. Full spectra and expanded sections (07–1.1 and 6.6–7.5 p.p.m.) of1H NMR spectra acquired using (a) 1-D1H NMR, (b) CPMG spin-echo pulse sequence and (c) by projecting the acquired 2-DJRES (pJRES). Spectra were acquired on CCRF-CEM leukaemia cells treated with solvent control (Control), Dex (50 nM), DCA (20 mM), RAP (100 nM) Vin (1 nM) and asparaginase at three different doses (A1, 1 U ml−1; A01, 0.1 U ml−1; A001, 0.01 U ml−1) following cell lysis and metabolism inactivation via addition of SDS and ultrasonication. The spectra acquired using the aforementioned pulse sequences show important alterations on the resonance intensities of selected metabolites (Ile, isoleucine; Leu, leucine; Val, valine; Tyr, tyrosine, His histidine; Phe, phenylalanine) as highlighted by the PCA scores plots obtained from analysis of spectra acquired using (d) 1-D (PC1 versus PC3), (e) CPMG (PC1 versus PC3) and (f)JRES pulse sequences (PC1 versus PC2) on CCRF-CEM cells with and without drug treatments. 2b ) and two-dimensional (2-D) 1 H J -resolved ( J RES; included in Figure 2c as 1-D projections of 2-D J RES spectra, p J RES) sequences. The enlarged sections (0.7–1.1 and 6.6–7.5 p.p.m.) of 1 H NMR spectra acquired on CCRF-CEM cells using the aforementioned techniques, highlight the efficacy of relaxation-edited CPMG and p J RES pulse sequences in removing the residual broad signals from cell debris including macromolecules (for example, proteins and lipoproteins). This enables identification and relative quantification of small metabolites in both the aliphatic and in the aromatic regions of the spectra (for example, valine, leucine, tyrosine) without the need of centrifugation steps. In addition, p J RES spectra provide proton-decoupled NMR spectra useful for reducing congestion and increasing metabolite specificity. Similar groupings and separation among all the eight treatments (six replicates per treatment) were observed comparing the PCA scores plots (PC1 and PC3) of CCRF-CEM leukaemia cells of 1D ( Fig. 2d ) and CPMG spectra ( Fig. 2e ). The PCA scores plots (PC1 and PC2), obtained using J RES pulse sequence ( Fig. 2f ), show an excellent separation and superior groupings for all the treatments compared with the scores plots using the other two techniques. Figure 2: Comparison of different NMR pulse sequences. Full spectra and expanded sections (07–1.1 and 6.6–7.5 p.p.m.) of 1 H NMR spectra acquired using ( a ) 1-D 1 H NMR, ( b ) CPMG spin-echo pulse sequence and ( c ) by projecting the acquired 2-D J RES (p J RES). Spectra were acquired on CCRF-CEM leukaemia cells treated with solvent control (Control), Dex (50 nM), DCA (20 mM), RAP (100 nM) Vin (1 nM) and asparaginase at three different doses (A1, 1 U ml −1 ; A01, 0.1 U ml −1 ; A001, 0.01 U ml −1 ) following cell lysis and metabolism inactivation via addition of SDS and ultrasonication. The spectra acquired using the aforementioned pulse sequences show important alterations on the resonance intensities of selected metabolites (Ile, isoleucine; Leu, leucine; Val, valine; Tyr, tyrosine, His histidine; Phe, phenylalanine) as highlighted by the PCA scores plots obtained from analysis of spectra acquired using ( d ) 1-D (PC1 versus PC3), ( e ) CPMG (PC1 versus PC3) and ( f ) J RES pulse sequences (PC1 versus PC2) on CCRF-CEM cells with and without drug treatments. Full size image We also performed pairwise PCAs comparing each of the drug treatments to the control samples. The percent variability obtained from these analyses (PC1 and PC2) and the multivariate Z -factor ( Supplementary Methods ) values ( Supplementary Table S2 ) show again the benefits of J RES in particular for Dex and Vin drug treatments. These differences of J RES can be in part attributed to a smaller number of variables, due not only to simplification of the spectra by decoupling of the multiplets but also to the reduced sensitivity, due to smaller number of scans in direct dimension, compared with 1-D and CPMG techniques. The loadings plot ( Fig. 1e ) indicates the weighting to the first component of the PCA score plot ( Fig. 1d ) of different spectral bins; in a similar manner, we have introduced Z -factor values at each bin of the NMR spectra ( Supplementary Methods ). The Z bin -values, superimposed to the loadings plots for each comparison of control and individual drug intervention ( Fig. 1e ), indicate that treatment with DCA-induced relevant metabolic changes (for example, pyruvate, glutamate, lactate) characterized by Z bin -factor values greater than 0.2 satisfying the requirements for a high-throughput assay [15] . To test the general applicability of high-content NMR-based metabolomic screening, we delivered the same drug treatments administered to non-adherent CCRF-CEM cells to the adherent ovarian SKOV-3 cells, a more drug-resistant mammalian cell line. As expected, the responses to drugs treatments in SKOV-3 cells were less pronounced compared with CCRF-CEM cells, as indicated by the smaller percent variation of the first and second principal components ( Fig. 3a ). However, the observed metabolic variations ( Fig. 3a ) support the applicability of this approach also to drug resistant and adherent cell lines. 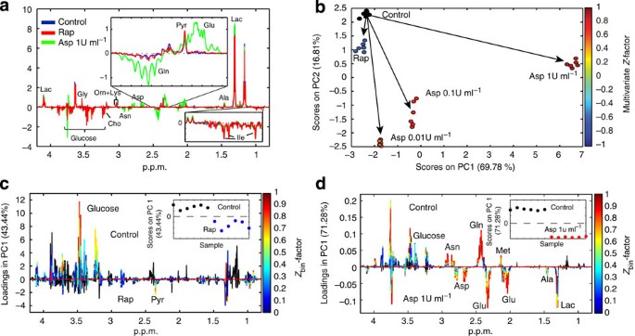Figure 3: NMR-based metabolomic screening of drug treatment in AML primary cells. (a) Difference spectra obtained by subtracting the average NMR spectrum of the medium, incubated without the cells in the 96-well plate subtracted from the average NMR spectra of AML primary cells with and without 24 h of 100 nM Rap or 1 U ml−1Asp drug treatment. (b) PCA scores plot (PC1 versus PC2) colour-coded according to the multivariateZ-factor values for each treatment group (Rap (Z=−0.90), A1 (Z=0.83), A01 (Z=0.77) and A001 (Z=0.42)). (c,d) PCA loadings plots and the superimposedZbin-values identify both the contribution and theZ-factor values of each bin of NMR spectra from a pairwise comparison of control and drug intervention (c) RAP and (d) Asparaginase treatments. Ile, isoleucine; Lac, lactate; Ala, alanine; Glu, glutamate; Pyr, pyruvate; Gln, glutamine; Asp, aspartate; Asn, asparagine; Orn, ornithine; Lys, lysine; Cho, choline; Gly, glycine. Figure 3: NMR-based metabolomic screening of drug treatment in AML primary cells. ( a ) Difference spectra obtained by subtracting the average NMR spectrum of the medium, incubated without the cells in the 96-well plate subtracted from the average NMR spectra of AML primary cells with and without 24 h of 100 nM Rap or 1 U ml −1 Asp drug treatment. ( b ) PCA scores plot (PC1 versus PC2) colour-coded according to the multivariate Z -factor values for each treatment group (Rap ( Z =−0.90), A1 ( Z =0.83), A01 ( Z =0.77) and A001 ( Z =0.42)). ( c , d ) PCA loadings plots and the superimposed Z bin -values identify both the contribution and the Z -factor values of each bin of NMR spectra from a pairwise comparison of control and drug intervention ( c ) RAP and ( d ) Asparaginase treatments. Ile, isoleucine; Lac, lactate; Ala, alanine; Glu, glutamate; Pyr, pyruvate; Gln, glutamine; Asp, aspartate; Asn, asparagine; Orn, ornithine; Lys, lysine; Cho, choline; Gly, glycine. Full size image We believe that the applicability of high-content NMR-based metabolomic screening might be extended also to other types of intervention such as miRs treatments. Indeed, the extent of the metabolic responses in human cell lines following transfection of miRs is not known [16] . Therefore, we tested whether the sensitivity of our HCS method was sufficient to detect metabolic changes in HeLa cells transfected with mir-121 and mir-16. We used premiRs as negative controls, which are chemically modified double-stranded RNA molecules designed to mimic endogenous miR molecules ( Supplementary Methods ). These miRs were selected because they were computationally predicted to target multiple metabolic enzymes. We found that the developed method was capable of detecting metabolic perturbation induced by miRs treatments as observed by the PCA scores plots (PC1 and PC2) and the multivariate Z -factor values ( Fig. 3b ). More specifically, mir-16 induced a more pronounced metabolomic alteration on HeLa cells compared with mir-121. Metabolomic NMR-based drug screening in acute myeloid leukaemia (AML) primary cells Owing to the small amount of cells required for our high-throughput metabolomic screening method, we believe that this procedure could be valuable to study the response to treatment in primary cells, while avoiding phenotypic changes induced by growth in culture. Cells isolated from bone marrow specimens of an untreated AML patient were treated for 24 h with Rap and L -asparaginase at different doses. Following treatment, the samples were prepared for the NMR analysis as detailed above. To emphasize the metabolic changes in the primary cell samples after the 24 h of treatment, we subtracted the NMR spectra acquired on unconditioned medium (incubated without cells in the same 96-well plate; Fig. 1a ) from those acquired on AML primary cells with and without drug intervention (for example, L -asparaginase 1 U ml −1 , Fig. 4a ). The difference spectra clearly indicated distinct changes in the metabolome of primary cells, including changes in isoleucine, alanine and ornithine. An unsupervised multivariate analysis was then performed on the acquired 1 H NMR spectra ( Fig. 4b ). PCA scores plots (PC1 and PC2) and related multivariate Z -factor values for Rap ( Z =−0.90), A1 ( Z =0.83), A01 ( Z =0.77) and A001 ( Z =0.42) confirm that different responses of primary cells to the drug treatments are detected ( Fig. 4b ). The overall response of AML primary cells to treatment was limited for Rap treatment (as observed from the negative multivariate Z -factor values), and increasingly more pronounced following treatment with increasing doses of L -asparaginase. In addition, for Rap treatment few metabolic changes (for example, pyruvate and glucose) had Z bin -factor values greater than 0.5 ( Fig. 4c ). This point-by-point analysis of Z -values for the L -asparaginase treatment indicated that besides the metabolites directly affected by the enzymatic activity of L -asparaginase (that is, asparagine and glutamine [17] , [18] ), other compounds, including glucose, lactate, alanine and methionine, were affected by this drug intervention ( Fig. 4d ). 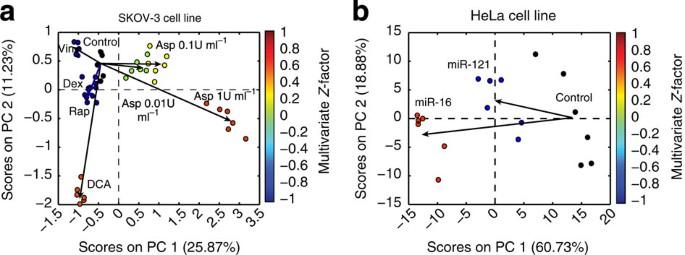Figure 4: High-content NMR-based metabolomic screening in adherent cell lines. PCA scores plots (PC1 versus PC2) obtained from the analysis of the1H-NMR spectra of (a) human ovarian carcinoma cell line (SKOV-3) after 24 h of treatment with different types of drugs and (b) human epithelial carcinoma cell lines (HeLa) after 24 h of miRs (miR-16 and miR-121) treatment. Each treatment-group on the PCA scores plots is colour-coded according to the multivariateZ-factor value (colour bar) obtained from the pairwise PCA comparison of treatment versus control for SKOV-3 (Dex (Z=−5.83), DCA (Z=0.45), Rap (Z=−3.07), Vin (Z=−1.84 ), A1 (Z=0.70), A01 (Z=0.01), A001 (Z=0.24)) and HeLa (mir-16 (Z=0.34) and mir-121 (Z=−0.55)) cell lines. Figure 4: High-content NMR-based metabolomic screening in adherent cell lines. PCA scores plots (PC1 versus PC2) obtained from the analysis of the 1 H-NMR spectra of ( a ) human ovarian carcinoma cell line (SKOV-3) after 24 h of treatment with different types of drugs and ( b ) human epithelial carcinoma cell lines (HeLa) after 24 h of miRs (miR-16 and miR-121) treatment. Each treatment-group on the PCA scores plots is colour-coded according to the multivariate Z -factor value (colour bar) obtained from the pairwise PCA comparison of treatment versus control for SKOV-3 (Dex ( Z =−5.83), DCA ( Z =0.45), Rap ( Z =−3.07), Vin ( Z =−1.84 ), A1 ( Z =0.70), A01 ( Z =0.01), A001 ( Z =0.24)) and HeLa (mir-16 ( Z =0.34) and mir-121 ( Z =−0.55)) cell lines. Full size image High-content NMR-based metabolomic screening of KI library Protein kinases control a wide range of cellular processes including cell metabolism [19] , [20] . Therefore, monitoring cell metabolism during treatment is extremely valuable to investigate the cellular response and treatment efficacy, in particular, as an evaluation criterion complimentary to standard screening methods. As a first application, here we applied the high-content NMR-based metabolomic screening combined with the ATP assay to monitor the cellular metabolomic response for a library of KIs ( Supplementary Table S4 ). We first used the ATP bioluminescence measurements to investigate changes in CCRF-CEM cell viability following treatment with approximately 250 KIs at 24 and 72 h. We then selected 56 KIs based on ATP values showing very low to moderate changes. Compounds causing very pronounced changes in viability after 24 h were excluded. Cell viability measurements ( Fig. 5a ) and the NMR-based metabolomic screening were performed after 24 h of treatment with 56 KIs in CCRF-CEM cells (in triplicates). We calculated the multivariate Z -factor for each KI treatment ( Fig. 5b ), and for a subset of metabolites we determined the Z bin -values ( Fig. 5c ) and their relative concentration (as a percent of control; Fig. 5d ). Several metabolic changes induced by the drugs were clearly correlated ( Supplementary Figure S6 ). 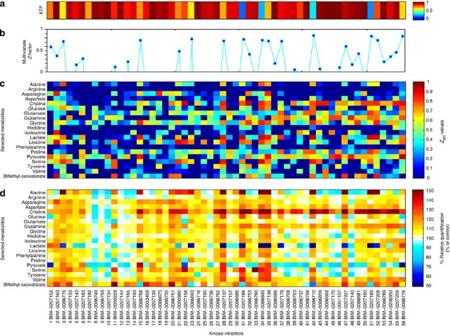Figure 5: NMR-based metabolomic screening of a library of KIs. (a) ATP assay was used to measure the cell viability of CCRF-CEM cells following 24 h of treatment with 56 KIs (1–56 BIM). The final concentration of each drug treatment was 1 μM. The mean luminescence values of cells treated with KI were normalized to the average ATP value for untreated cells (solvent control). (b) Principal component analysis was performed on the1H NMR spectra acquired in triplicates and a multivariateZ-factor value was calculated for each KI. For a subset of all the observed metabolites we determined theZbin-values (c) and their relative concentration (d, as percent of control). Figure 5: NMR-based metabolomic screening of a library of KIs. ( a ) ATP assay was used to measure the cell viability of CCRF-CEM cells following 24 h of treatment with 56 KIs (1–56 BIM). The final concentration of each drug treatment was 1 μM. The mean luminescence values of cells treated with KI were normalized to the average ATP value for untreated cells (solvent control). ( b ) Principal component analysis was performed on the 1 H NMR spectra acquired in triplicates and a multivariate Z -factor value was calculated for each KI. For a subset of all the observed metabolites we determined the Z bin -values ( c ) and their relative concentration ( d , as percent of control). Full size image To confirm some of the hits of the first metabolomic screen ( Fig. 5 ), nine KIs were chosen for a secondary screen ( Supplementary Figs S7–S9 ). Four of the repeated compounds were selected because of the action on a well-known clinical phenotype, the lactate/pyruvate ratio ( Fig. 6a–d ). Five more compounds were chosen to provide additional data on measurement reproducibility. The results of the second screen ( Supplementary Fig. S7a,b ) were consistent with the first assay and the average coefficient of variation in metabolite changes between the two screens was 0.09±0.01 (mean±s.e.m.). Most of the metabolites showed comparable changes in the two screenings ( Supplementary Fig. S7c,d ). The second screen was also performed on CCRF-CEM cells treated using a 10-fold lower dose of KIs (0.1 μM; Supplementary Fig. S8 ). Most low-dose treatments did not affect the ATP cell viability; however significant metabolic alterations were observed for some treatments (for example, BIM-00866768 and BIM-0086776; Supplementary Fig. S8 ). To confirm the observed results, hit follow-up dose–response experiments were performed using six different concentrations [21] of KI in the range of 0.05–2 μM ( Supplementary Fig. S9 ). These concentrations were chosen with the intent of investigating the metabolomic response of CCRF-CEM cells to KI treatment without affecting their cell biomass. IC50 values were calculated based on the 50% reduction of ATP levels induced by treatment ( Supplementary Table S5 ). 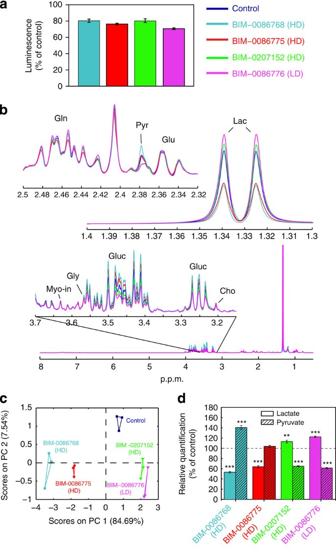Figure 6: Metabolic modulation induced in CCRF-CEM cells by four KI hits. Four KIs found to cause similar drop (by ~20%) of ATP values in CCRF-CEM cells selected. The drugs eEF-2 KI (BIM-0207152), MK2 inhibitor (BIM-0086775) and an inhibitor of PKA, PKC and PKG (BIM-0086768) were administered at the high dose (1 μM), and NF-KB activation inhibitor (BIM-0086776) at low dose (0.1 μM). (a) ATP assay (as % of control) following KI treatments is reported as the mean values (bars) ±s.e.m. (error bars;N=3). (b) Representative sections of average1H NMR spectra acquired on CCRF-CEM cells with and without KI treatment are expanded (Gln, glutamine; Pyr, pyruvate; Glu, glutamate; Cho, choline; Gluc, glucose; Gly, glycine; Myo-in, myo-inositol). (c) Principal component analysis (PC1 versus PC2) was performed on the1H NMR spectra of treated and untreated CCRF-CEM cells acquired in triplicates. (d) Relative concentrations of lactate and pyruvate calculated as percent of control are reported as the mean values (bars)±s.e.m. (error bars;N=3). Statistical comparison between data obtained from untreated and KIs treatment was performed using an unpaired Student'st-test (statistical significance: **P<0.01 and ***P<0.001). Figure 6: Metabolic modulation induced in CCRF-CEM cells by four KI hits. Four KIs found to cause similar drop (by ~20%) of ATP values in CCRF-CEM cells selected. The drugs eEF-2 KI (BIM-0207152), MK2 inhibitor (BIM-0086775) and an inhibitor of PKA, PKC and PKG (BIM-0086768) were administered at the high dose (1 μM), and NF-KB activation inhibitor (BIM-0086776) at low dose (0.1 μM). ( a ) ATP assay (as % of control) following KI treatments is reported as the mean values (bars) ±s.e.m. (error bars; N =3). ( b ) Representative sections of average 1 H NMR spectra acquired on CCRF-CEM cells with and without KI treatment are expanded (Gln, glutamine; Pyr, pyruvate; Glu, glutamate; Cho, choline; Gluc, glucose; Gly, glycine; Myo-in, myo-inositol). ( c ) Principal component analysis (PC1 versus PC2) was performed on the 1 H NMR spectra of treated and untreated CCRF-CEM cells acquired in triplicates. ( d ) Relative concentrations of lactate and pyruvate calculated as percent of control are reported as the mean values (bars)±s.e.m. (error bars; N =3). Statistical comparison between data obtained from untreated and KIs treatment was performed using an unpaired Student's t -test (statistical significance: ** P <0.01 and *** P <0.001). Full size image Four of the nine KIs considered above were then chosen, selecting the compounds inducing moderate ATP level drops to prevent relevant changes in cell biomass. These four KIs reproducibly affected the relative concentrations of lactate and pyruvate in opposite directions ( Figs 5 and 6 ; Supplementary Figs S7–S9 ). An eEF-2 KI (BIM-0207152), and a NF-κB activation inhibitor (BIM-0086776) increased lactate/pyruvate ratio ( Fig. 6d ), whereas an MK2 inhibitor (BIM-0086775), and an inhibitor of PKA, PKC and PKG (BIM-0086768) induced a decrease. Concurrently, mild and comparable effects on ATP levels were observed, consistent with reduced cell proliferation ( Fig. 6a ). Moreover, these inhibitors were not identical in their action in fact engendered distinct metabolic changes, including glucose, alanine, serine, choline and glutamine ( Fig. 6b ). Multivariate statistical analysis ( Fig. 6c ) indicates that BIM-0207152 and BIM-0086776 induced similar alterations in cellular metabolic profiles, different from those induced by BIM-0086775 and BIM-0086768, and distinct from untreated controls. The two inhibitors (BIM-0207152 and BIM-0085776) that induce similar metabolic modulations in CCRF-CEM cells ( Fig. 6 ) also show similar responses in cell survival of primary cells from acute leukaemia patients. Preliminary results from four leukaemia patients indeed showed a high correlation in the individual response between these two drugs after 24 h in culture ( Supplementary Fig. S10 ). Cultured cell lines are well-established models for the study of cancer [22] , [23] , [24] . Despite the numerous in vitro and ex vivo studies, a high-content metabolomic assay for screening drug libraries using mammalian cells has not been reported. The methodology developed in this work describes an innovative approach using NMR-based metabolomics for drug screening. The rationale for using NMR as the platform of choice was dictated by the ability of this analytical technique to handle samples containing complex and relatively unrefined mixtures of compounds. More specifically, the samples considered in this study required only minimal sample preparation without the need of additional separation or filtration step (for example, proteins removal). Furthermore advantageous are the low experimental variability and reasonable cost per sample. The main drawback associated with the use of NMR is the relatively limited number of compounds that can be detected. Owing to this limitation, our metabolomic HCS method do not provide metabolic profiles as those described by us and others using more in-depth metabolomic techniques [8] , [11] , [21] , [22] , [25] , [26] , [27] , [28] . Nevertheless, the assay we describe is suitable for a high-throughput primary screen, and should be followed, as it is commonly the case, by secondary assays analysing the exo- and endo-metabolomes of selected hits likely using a combination of different analytical platforms [8] , [11] , [21] , [22] , [25] , [26] , [27] , [28] . Other techniques including turbulent flow chromatography interfaced with MS might represent a valid tool for a metabolomic screening capable of increasing the number of identified metabolites compared with NMR techniques [29] , with additional sample preparation steps. Although not comprehensive of all metabolites, the wealth of information obtained from the multivariate metabolic readout is of great advantage for drug screening purposes. In fact, although most primary drug screens on mammalian cells are based on single readout, high-content metabolomic screening allows the parallel measurements of an array of metabolites and is designed to provide additional valuable information and criteria for the selection of the most effective individual or combinatorial drug interventions. To allow the rapid preparation and metabolomic screening of hundreds of samples, we validated a novel protocol for lysing the cells and immediately quenching cellular metabolism, using SDS, a powerful denaturating detergent widely used in protein biochemistry [30] , and in micelle-assisted diffusion-ordered spectroscopy for stereoisomer resolution [31] . The content of a single well from a 96-well plate was used for the assay without the need of pooling the content of several wells, enabling maximized yield per plate. Moreover, the sensitivity of our high-content metabolomic screening method was proven adequate to monitor metabolic perturbations induced by drug intervention in both cultured cell lines and in AML primary cells as well as following treatment with miRs. The metabolomic study of miRs could potentially be extended to the entire set all known human miRs (around 500), and therefore contribute to the understanding of this complex intracellular regulatory system. Altogether, using our approach, hundreds of samples can metabolically be inactivated in ~5 min and a metabolomic screening of around 100 samples can be performed in 24 h. Progress in NMR spectroscopy, for example, in probe hardware design, will increase the sensitivity of this method and allow the applicability to volumes obtained from higher density plates (for example, 384-well plates). In particular, the relatively new area of microprobe and multiple coil probeheads shows great promises for high-throughput NMR experiments [32] . In the area of NMR data processing, continuous efforts are devoted to the development of new algorithms for reducing multiple readout parameters and automating identification and quantification of metabolites [33] . Here we capitalized on NMR pulse sequences (CPMG and J RES), which warrant highly reproducible analyses of small molecules even in the presence of residual proteins or cell debris in the sample. Multivariate Z -factor values derived from PCA were used to evaluate the quality of the NMR-based metabolomic screening assay. Furthermore, because NMR spectra produce arrays of complex data (as opposed to a single outcome), we also introduced the Z bin -value as a localized parameter assessing the effect of drug treatment on each metabolite. Since the development of imatinib (known as CGP 57148 (ref. 34 ) and subsequent application for treatment of chronic myeloid leukaemia, KIs have received increasing attention as anticancer drugs. Activation of oncogenic pathways including PI3K/AKT/mTOR, involved with altered bioenergetic pathways, such as glycolysis, fatty acid and glutamine metabolisms, has suggested novel targets for cancer treatment [23] , [24] , [27] , [35] , [36] . Therefore, monitoring cell metabolism during treatment is extremely valuable to investigate cellular response and treatment efficacy. Here we screened a library of KIs and shown different metabolic adaptations following 24 h of treatment. Metabolomic data showed that inhibitors could modulate metabolic substrates uptake and product excretion in the presence of similar ATP levels. In our first application, we focused on four KIs that can change the lactate/pyruvate ratio, an important and clinically validated measure of the intracellular redox potential and of cellular respiration [37] , [38] . The lactate/pyruvate ratio is a potential therapeutic target relevant not only to hypoxic and ischaemic disease but also to many other pathologies, including genetic mitochondrial diseases [37] , [38] . The focus on compounds functioning on this important parameters emerged after the first screen, demonstrating one advantage (hypothesis generation) of the metabolomic method we describe as compared with drug screens based on the measurement of one or two metabolites. There are many other possible applications of this method, for example lactate production and substrate utilization in cancer versus non-cancer cells [24] , [36] or gluconeogenesis from different substrates in hepatocytes, relevant to diabetes [39] , [40] . Importantly, because the measurements are performed within a global metabolic profile, they can also provide a series of compounds with partially different mechanisms of actions, which can be explored for potential synergies [41] , [42] , [43] , [44] . Because the inhibitors we used have known targets, the screen can also be used to generate hypotheses about metabolic relevant signal transduction mechanisms. For example, the two most closely related KIs ( Fig. 4c ) target eEF-2 kinase [45] and NF-kB [46] . In addition, eEF-2 kinase has been linked to other metabolically relevant pathways and to the autophagic process [47] . These relationships can be followed up experimentally, with the caveat that we might not know all the targets of the inhibitors we have used. We believe that this NMR-based assay might find an immediate relevant application for screening a large number of individual or combinatorial drug interventions reducing the number of possible drugs to be studied more in detail. In addition, it might find an immediate relevant application into clinical studies. The possibility of using cells directly taken from patients might open new routes for the development of personalized drug treatment [48] , [49] . Primary AML cells and cell lines Bone marrow specimens from untreated AML and lymphoblastic leukaemia patients were obtained from the Rady Children's hospital. Informed consent was obtained from all patients involved and study was performed in accordance with the Institutional Review Board guidelines. Within 6 h after sampling, mononuclear cells were isolated by Ficoll-paque (GE Healthcare) density gradient centrifugation (1.077 g cm −3 ) at 400 g for 30 min followed by three washes in PBS. Isolated mononuclear cells were allowed to adhere to the 96-well plate overnight in RPMI 1640 medium (HyClone). Non-adherent mononuclear cells were collected to enrich lymphocyte population. CCRF-CEM and SKOV-3 cell lines were maintained in exponential proliferation in RPMI 1640 medium (HyClone), whereas HeLa cells were grown in DMEM (HyClone). Both media were supplemented with 10% FBS (HyClone), 1% 200 mM L -glutamine (Omega) and 1% penicillin/streptomycin (Omega). The cells were cultured in a humidified chamber at 37 °C with 5% CO 2 . Isolated non-adherent mononuclear, CCRF-CEM, SKOV-3 and HeLa cells were seeded in 96-well plates (Greiner Bio One) at the density of 3×10 5 , 1×10 5 , 3×10 4 , 1.5×10 4 cells per well, respectively, and allowed to adapt/attach for 6 h before treatment. Doubling time was 24, 48 and 24 h for CCRF-CEM, SKOV-3 and HeLa cells, respectively. For each cell type, the number of cells seeded per well was determined using a luminescent ATP-detection assay (Perkin Elmer; Supplementary Methods ) such that the cells remained in their linear range of growth and the maximum number of cells per well was obtained 30 h after seeding (accounting for 6 h of adaptation and 24 h of treatment). Drug treatments Both CCRF-CEM and SKOV-3 cells were treated for 24 h with the following drugs: DCA (20 μM; Sigma-Aldrich), Dex (50 nM, Calbiochem), Rap (100 nM; Sigma-Aldrich), Vin (1 nM; Sigma-Aldrich) and three different concentrations of L -asparaginase (0.01, 0.1, 1 U ml −1 ; BioVendor Inc.). An untreated control group (solvent control) was also included in all the assays. All the drug treatments were performed in six replicates per condition. No alterations in cell numbers were observed following 24 h of drug treatment. To reduce bias, the treatments were administered based on a randomized list of well positions. Sample preparation for HCS experiments The cells of interest were seeded in a 96-well plate with 200 μl of appropriate medium. A total volume of 10 μl of SDS was added to the culture medium via a multichannel electronic pipette. The final concentration of SDS in each well was 0.5% w/v, unless otherwise noted (all experiments with the exception of the optimization procedure detailed below). Immediately after addition of SDS, the 96-well plates were sealed and sonicated in an ice-cold ultrasonicating water bath for 5 min. The water bath temperature at the beginning of sonication was 4 °C and during sonication never exceeded 6 °C. At the end of sonication 160 μl was transferred from each well into a 3-mm NMR tube (Norell) containing TMSP-d4 (Cambridge Isotope Laboratories; final concentration 0.5 mM), phosphate buffer (final concentration 100 mM) and 10% of D 2 O (Cambridge Isotope Laboratories) to obtain a total volume of 200 μl. The overall time between dispensing SDS to the 96-well plate and sonicating the entire content of the well for lysing the cells and quenching their enzymatic activity was approximately 5 min. NMR experiments One-dimensional standard 1 H NMR and CPMG and 2-D 1 H J RES spectra were acquired on 500-MHz Bruker and 600-MHz Bruker Avance equipped with a TCI cryoprobe spectrometers (Bruker BioSpin Corp.), both equipped with an autosampler at 30 °C [50] , [51] , [52] . All the pulse sequences were implemented with excitation sculpting to suppress the water signal [53] . One-dimensional and CPMG spectra were acquired using a 90° flip angle, 6 kHz spectral width, relaxation delay of 1 s, 16k data points, 8 dummy scans and 256 or 512 transients (approximately 15 or 30 min of acquisition per sample). Spin-spin relaxation delay of CPMG was set to 100 ms. Double spin-echo sequence suppressing strong coupling artifacts was used to acquire 2-D J RES spectra [52] . Thirty-two increments were recorded in the indirect dimension using 16 transients per increment, 16k data points with 8 dummy scans and a recycle delay of 2 s; spectral widths of 6 kHz and 50 Hz were set in direct and indirect dimension, respectively, (~45 min of acquisition per sample). Before Fourier transformation, 1-D and CPMG spectra were zero-filled and processed by multiplying the free induction decay by an exponential line broadening function of 0.5 Hz. Before Fourier transformation, 2-D J RES spectra were zero-filled in both dimensions, and apodization using combined sine-bell/exponential window function in the direct dimension and by a sine-bell function in the incremented dimension has been applied [54] . Following Fourier transformation, the magnitude mode spectra were tilted by 45°, symmetrized and skyline projected (p J RES). All the NMR data sets were processed using NMRLab [55] in the MATLAB programming environment (MathWorks, Inc.). Post processing of NMR spectra included scaling according to the probabilistic quotient method [56] , alignment, exclusion of selected signals arising from solvents, TMSP and DCA, binning at 0.005 p.p.m., and application of a generalized log transformation [57] . NMR resonances of metabolites were assigned using the Chenomx NMR Suite (version 6.0; Chenomx Inc.) and other available libraries [58] , [59] . Optimization and validation of metabolomics HCS method To optimize the amount of SDS required to completely quench cell metabolism we monitored residual cell viability and metabolic activity in samples prepared without or with various amounts of SDS. Ten different concentration of SDS were considered ranging between 0.01 and 2% w/v (final concentration per well). Cellular viability and residual metabolism were monitored using both ATPlite assay ( Supplementary Methods ) and cell count (Countess automated cell counter, Invitrogen) measurements in samples prepared using ultrasonication and with and without the addition of SDS. All the measurements were performed with six replicates per condition. Furthermore, to check for residual metabolism, a series of 1-D NMR spectra were collected every 30 min over a period of 8 h for live CCRF-CEM cells, cell lysed using only ultrasonication and cells simultaneously lysed and SDS inactivated. Subsequent multivariate analysis (PCA) was performed on 16 spectra per condition. For these experiments, the NMR spectra were acquired at 37 °C to maintain more suitable conditions for live cells. To further validate the sample preparation method developed and assess a possible metabolomic bias arising from plate-to-plate variability, we acquired 1-D 1 H-NMR spectra of six wells per plate and per treatment condition over five different plates (in total 60 1 H-NMR spectra, 30 replicates per condition) for CCRF-CEM cells with and without 1 U ml −1 L -asparaginase treatment. Screening of KIs library Fifty-six KIs from the 384-well protein KI library I (InhibitorSelect, EMD Chemicals Inc.; Supplementary Table S4 ) were dissolved in dimethylsulphoxide, administered to CCRF-CEM cells at 1 μM (final concentration) for 24 h and luminescence and NMR experiments were performed at least in triplicates. NMR spectra of the medium, containing solvent control and incubated with and without the cells in the same 96-well plate, were acquired in triplicates. To confirm initial hits, nine KIs were chosen, and ATP assay and NMR experiments were acquired for three or more independent repeats on CCRF-CEM cells following 24 h of treatment of KI at two different doses. For every plate, NMR spectra of two different controls, cells receiving solvent control and media incubated in the same 96-well plate without the cells but containing solvent control were acquired as well. The drugs were eEF-2 KI (BIM-0207152), 5-iodo-indirubin-3′-monoxime (BIM-0207163), MK2a inhibitor (BIM-0086775), ERK inhibitor II (BIM-0086749), PKC inhibitor (BIM-0050229), K-252a, Nocardiopsis sp. (BIM-0086768), Fascaplysin, Synthetic (BIM-0086751), Wee1 inhibitor II (BIM-0207209) and NF-KB activation inhibitor (BIM-0086776) all administered at 1 μM (high dose) and 0.1 μM (low dose). Hit follow-up studies were performed using dose–response experiments for the abovementioned nine KIs. Dose–response experiments were performed treating CCRF-CEM cells using six different clinically relevant concentrations of KI in the range of 0.05–2 μM. The intent of our study was to investigate the metabolomic response to KI treatment without affecting the cell biomass. IC50 values were calculated ( Supplementary Table S4 ) based on the 50% reduction of ATP levels induced by treatment. No alterations in cell numbers were observed after 24 h induced by KI treatments. Statistical and chemometric analysis After processing, NMR spectra were mean-centered and then subjected to PCA [60] using MATLAB. Multivariate Z -factor values were calculated as indicated in Supplementary Equations S1-S2 (refs 13 , 15 ; Supplementary Methods ). The relative concentrations of selected metabolites (as percent of control) are reported as mean values±s.e.m Statistical comparison between data obtained from untreated and individual KIs treatment was performed using an unpaired Student's t -test (statistical significance: * P <0.05, ** P <0.01 and *** P <0.001). How to cite this article: Tiziani, S. et al . Metabolomic high-content nuclear magnetic resonance-based drug screening of a kinase inhibitor library. Nat. Commun. 2:545 doi: 10.1038/ncomms1562 (2011).